Identification and characterization of a multidomain hyperthermophilic cellulase from an archaeal enrichment Despite extensive studies on microbial and enzymatic lignocellulose degradation, relatively few Archaea are known to deconstruct crystalline cellulose. Here we describe a consortium of three hyperthermophilic archaea enriched from a continental geothermal source by growth at 90 °C on crystalline cellulose, representing the first instance of Archaea able to deconstruct lignocellulose optimally above 90 °C. Following metagenomic studies on the consortium, a 90 kDa, multidomain cellulase, annotated as a member of the TIM barrel glycosyl hydrolase superfamily, was characterized. The multidomain architecture of this protein is uncommon for hyperthermophilic endoglucanases, and two of the four domains of the enzyme have no characterized homologues. The recombinant enzyme has optimal activity at 109 °C, a half-life of 5 h at 100 °C, and resists denaturation in strong detergents, high-salt concentrations, and ionic liquids. Cellulases active above 100 °C may assist in biofuel production from lignocellulosic feedstocks by hydrolysing cellulose under conditions typically employed in biomass pretreatment. Cellulose is the most abundant biopolymer on earth [1] . The hydrolysis of cellulose and its use as a microbial growth substrate is ubiquitous, as the thousands of annotated cellulases in the CAZy database attest [2] , [3] , [4] . It is therefore surprising that the Archaea, whose members have exploited most of the available carbon and energy sources on Earth, have relatively few species known to deconstruct lignocellulosic biomass [5] . This is especially true of the hyperthermophilic archaea. There are 35 genera of archaea with hyperthermophilic species that employ a wide range of carbon and energy sources. To date, only one hyperthermophilic archaeon, Desulfurococcus fermentans , demonstrated growth on crystalline cellulose (filter paper) at an optimum temperature of 81 °C (ref. 6 ). The genome sequences of many species of hyperthermophilic archaea do encode endoglucanases, notably Pyrococcus and Sulfolobus spp. ; however, cellulase genes predicted from archaeal genomes are rarely reported, and even the predicted presence of these genes does not imply an ability to grow on cellulosic substrates. Additionally, cellulases from hyperthermophiles lack identifiable cellulose binding domains, in contrast to the cellulases produced by organisms like Trichoderma reesei [7] and Clostridium thermocellum [8] that can grow using cellulosic carbon sources. These species have large and diverse inventories of glycosyl hydrolases (GHs), including multicopy hemicellulose and cellulose degrading-enzymes with various carbohydrate-binding domains. These cellulose-binding domains can be added to hyperthermophilic cellulases to increase degradation by domain addition, gene shuffling and other strategies [1] , [9] . For example, by adding a thermostable chitin-binding domain to the Pyrococcus horikoshii endoglucanase (EGph), higher activities on crystalline substrates were achieved [10] . The tight structure of lignocellulose is primarily responsible for its inherent stability and strength but presents a barrier to efficient hydrolysis, a significant problem when considering lignocellulose for biofuel production. Consequently, cellulosic biomass must first be subjected to pretreatment to increase the accessible surface area, and undergo either chemical or enzymatic deconstruction to release sugars that can be subsequently fermented to biofuels. Generally, enzymatic deconstruction and hydrolysis occurs slowly under conditions typically around 50 °C and pH 5.0. The conditions of many pretreatment processes are much more extreme, employing high temperatures combined with low or high pH, or steam explosion, for chemical pretreatment of feedstocks [11] . Strategies for commercial depolymerization of cellulose combine physicochemical pretreatment (acid or base) and enzymatic hydrolysis [12] . Therefore, thermophilic cellulases have been targets of research to engineer durable enzymes that can withstand harsher conditions to minimize the cost and complexity of adjusting process conditions between pretreatment and hydrolysis. Given that no characterized hyperthermophilic archaeal species contain a minimum set of exo-, and endo-, hemicellulases required to grow on lignocellulose above 90 °C, isolating a single cellulolytic species could be problematic. Hence, we set out to reconstitute a consortium of hyperthermophiles that could deconstruct lignocellulosic biomass at 90 °C. Our hypothesis was that hyperthermophilic archaea could be enriched to grow on pulverized plant biomass and further characterized by metagenomic sequencing and enzyme characterization. Metagenomic analysis of the high temperature consortium resulted in a collection of many genes annotated as GHs, in which 12 were assigned to the closed genome of the major strain. The expression of a thermostable endoglucanase from one of these genes resulted in the identification of the most thermoactive cellulase characterized, to date. Moreover, this cellulase has a unique multidomain architecture not yet observed in hyperthermophilic cellulases. Enrichment and extraction of native protein The enrichment strategy to identify hyperthermophiles that could degrade cellulose provided a strictly anaerobic three-species consortium capable of growth on Miscanthus, filter paper, Avicel (microcrystalline cellulose), and carboxymethylcellulose (CMC) at 90 °C. 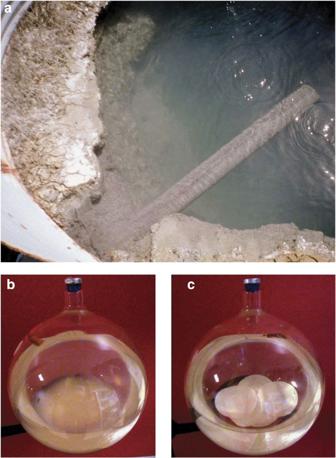Figure 1: Source of J1 enrichment and degradation of filter paper. (a) Source of the J1 enrichment. A circumneutral geothermal pool at 94 °C, with a level-maintaining syphon. Sediment from the floor of this site was enriched on pulverized Miscanthus at 90 °C and subsequently transferred to filter paper enriched media. (b) Degradation of filter paper by the J1 enrichment culture in a spherical 2 l culture flask. Circular discs of Whatman No. 3 filter paper were shredded and partially dissolved after incubation for 30 days at 90 °C. (c) Control Whatman No. 3 filter paper discs. Incubation as in panelb. Figure 1a shows the collection site of the sediment that produced the enrichment, a 94 °C geothermal pool in northern Nevada. Figure 1b shows the deconstruction of Whatman No. 3 filter paper by the J1 culture in a spherical growth flask, compared with an uninoculated control ( Fig. 1c ). See also Supplementary Fig. S1 . Repeated efforts to separate the individual species by decimal dilution and variation of growth conditions were unsuccessful. Hence, the consortium as a whole was analysed for potential cellulases of interest. Avicel was employed as the carbon source to identify the presence not only of excreted cellulases, but also to identify cellulases that are able to bind to an insoluble cellulolytic substrate. Such bound enzymes are considered to be a prerequisite for degradation of crystalline cellulose [1] , [5] . The consortium was scaled up to a 17.5-L batch culture and grown to mid-exponential phase. Cells and Avicel substrate were pelleted together by centrifugation and sonicated in buffer. The combined pellet was subjected to a series of four extractions in 0.6% (w/v) CHAPS detergent to remove insoluble membrane fractions and weakly bound proteins. Tightly bound proteins were eluted at 90 °C (1 h) with two extractions in 1% (w/v) CHAPS and 5% cellobiose. Additional protein was eluted with 1% SDS at 100 °C (15 min). The 1% CHAPS/5% cellobiose fraction showed detectable CMCase activity on zymograms. Active cellulases with apparent molecular weights of about 40 and 80 kDa were detected ( Fig. 2 ). Subsequent washes with 1% SDS at 100 °C yielded the release of additional hyperstable, high-molecular weight enzymes with CMCase activity, as indicated by the activity in a smaller number of more distinct bands with apparent molecular weights of about 80 and 180 kDa ( Fig. 2 ). It was apparent that this consortium was producing cellulases that could bind to Avicel particles and were able to withstand boiling in 1% SDS, abilities not yet observed in well-characterized cellulases from hyperthermophilic archaea. Therefore, metagenomics was used to identify potential cellulases from this consortium. Figure 1: Source of J1 enrichment and degradation of filter paper. ( a ) Source of the J1 enrichment. A circumneutral geothermal pool at 94 °C, with a level-maintaining syphon. Sediment from the floor of this site was enriched on pulverized Miscanthus at 90 °C and subsequently transferred to filter paper enriched media. ( b ) Degradation of filter paper by the J1 enrichment culture in a spherical 2 l culture flask. Circular discs of Whatman No. 3 filter paper were shredded and partially dissolved after incubation for 30 days at 90 °C. ( c ) Control Whatman No. 3 filter paper discs. Incubation as in panel b . 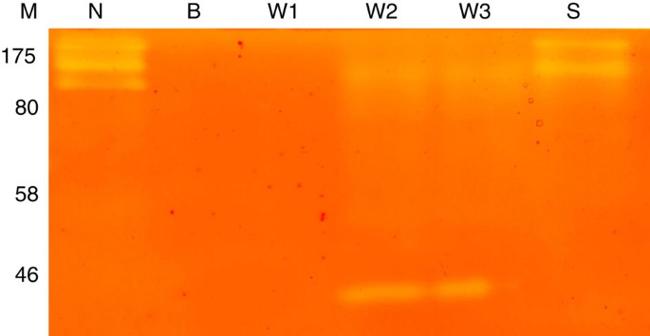Figure 2: Protein extraction and detection of CMCase activity. Protein extraction and detection of CMCase activity from proteins eluted from Avicel particles after deconstruction by J1 enrichment at 90 °C for 8 days. Image shows SDS–PAGE gradient zymogram, 10–15% acrylamide, with 0.2% CMC embedded in gel. Lanes: M-marker, N-native whole SDS extract, B-buffer only soluble extract, W1-0.6% CHAPS extract, W2-1% CHAPS 5% Cellobiose extract #1 (1 h incubation at 90 °C), W-3 1% CHAPS 5% Cellobiose extract #2 (1 h incubation at 90 °C), S-1% SDS extract final wash (15 min incubation 100 °C). For lanes B through S, the Avicel pellet was sonicated continuously for 2 min in the wash solution. Full size image Figure 2: Protein extraction and detection of CMCase activity. Protein extraction and detection of CMCase activity from proteins eluted from Avicel particles after deconstruction by J1 enrichment at 90 °C for 8 days. Image shows SDS–PAGE gradient zymogram, 10–15% acrylamide, with 0.2% CMC embedded in gel. Lanes: M-marker, N-native whole SDS extract, B-buffer only soluble extract, W1-0.6% CHAPS extract, W2-1% CHAPS 5% Cellobiose extract #1 (1 h incubation at 90 °C), W-3 1% CHAPS 5% Cellobiose extract #2 (1 h incubation at 90 °C), S-1% SDS extract final wash (15 min incubation 100 °C). For lanes B through S, the Avicel pellet was sonicated continuously for 2 min in the wash solution. Full size image Sequencing and phylogenetic analysis Pyrosequencing of the DNA extracted from cells grown on Avicel yielded 1,283,902 pyrosequencing reads with a total of 497,707,575 bases. Assembly and dereplication resulted in 6.95 Mb in scaffolds that differed in the read density per kb in the following ratio: 100:5:3. Three 16S ribosomal RNA genes were identified and the closest matches to characterized organisms were Ignisphaera aggregans DSM 17230 (95%), Pyrobaculum islandicum DSM 4184 (98%), and Thermofilum pendens Hrk (93%). 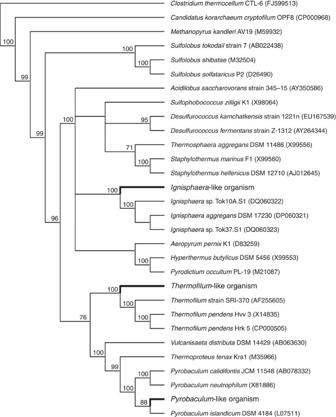Figure 3: Maximum likelihood phylogenetic tree. Maximum likelihood16S rRNA phylogenetic tree, showing the relationship of full-length 16S rRNAs from the three component organisms of the assembled metagenome. Branches in bold and labelled with larger type represent the three sequences from the metagenome. A maximum likelihood 16S rRNA gene phylogenetic tree is shown in Figure 3 . Similar topology and bootstrap supported was obtained for the Neighbour-joining method (results not shown) The 16S rRNA gene from the Ignisphaera -like organism was 99% identical to 16S rRNA clones from uncultured archaea from geothermal systems in both Nevada (accession number HM448083.1 ) and Montana (accession number EU635921.1 ). The Ignisphaera -like 16S rRNA (accession number JF509453 ) represented the dominant organism in the enrichment-based 16S rRNA clone libraries and on the large number of reads per kilobase of sequence ( ∼ 300) for 16S rRNA and the hyperthermophilic signature gene reverse gyrase, compared with read densities (<20) of these two genes from the other organisms. The genome of the dominant strain has recently been closed by additional Solexa (Illumina) sequencing using the same DNA sample, and assembled into a 1.92 Mb circular chromosome and a 21-kb circular plasmid. The reads associated with these scaffolds amount to 85.1% of the total Solexa generated database confirming that the Ignisphaera -like strain dominates the consortium. The metagenome is currently being annotated before submission in a subsequent paper. Figure 3: Maximum likelihood phylogenetic tree. Maximum likelihood16S rRNA phylogenetic tree, showing the relationship of full-length 16S rRNAs from the three component organisms of the assembled metagenome. Branches in bold and labelled with larger type represent the three sequences from the metagenome. Full size image Identification of carbohydrate-active enzymes Annotation analysis found a large number of GHs (37) and included 4 potential GH family 5 endoglucanases, based on automated annotation ( Supplementary Table S1 ). Twelve of these GHs were encoded by the closed genome of the dominant strain. One predicted GH, designated EBI-244 (accession number JF509452 ), was chosen for further study, because it was a potential multidomain cellulase, 842 amino acids in length, and a member of the TIM barrel glycosyl hydrolase superfamily (β/α) [8] . Large multidomain cellulases are ubiquitous amongst cellulolytic organisms but have not been previously found in hyperthermophilic archaea. The central domain of this enzyme (AA250-580) had a Pfam match ( E -value 1×10 −12 ) to the GH family 5 (GH5). The gene encoding EBI-244 was found on the chromosome of the dominant organism, and at 94 kDa, EBI-244 was the largest of three proteins encoded on the chromosome with Pfam hits to GH family 5 (GH5); the others were a 43 kDa Pfam match ( E -value 6.3×10 −67 ) and a 44 kDa Pfam match ( E -value 8×10 −52 ). According to BLASTp searches EBI-244 is a weak match to its closest apparent homologue, an uncharacterized hypothetical protein from Caldicellulosiruptor saccharolyticus (35% identity) ( Supplementary Fig. S3 ). The conserved central domain (AA250-580), indicated by dashed line in Supplementary Fig. S2 , had only 9 significant hits (NCBI nonredundant protein database) with BLAST E -values less than 1×10 −20 , including proteins from Herpetosiphon aurantiacus ATCC 23779, Spirochaeta thermophila DSM 6578, Spirochaeta thermophila DSM 6192, Opitutus terrae PB90-1, Chitinophaga pinensis DSM 2588, Zunongwangia profunda SM-A87, Clostridium leptum DSM 753, Victivallis vadensis ATCC BAA-548; with percent identities ranging from 25–35%. Sequence analysis of the EBI-244 enzyme Given the deduced size of this cellulase and the possibility of multiple domains beyond the standard GH domain, Hidden Markov model (HMM) methods were pursued to predict the domain architecture for EBI-244. On the basis of the scores and alignments from HMM analysis, the EBI-244 protein is predicted to encode four structural domains, with hydrophobic and Pro/Thr-rich regions at the amino terminus ( Fig. 4 ). The GH5 Pfam match was designated as domain 2 of EBI-244 and lies in the centre of the protein flanked by predicted structural domains on either side. Domains 1, 3 and 4 do not show similarity to any characterized domain or protein in the major databases (BLAST hits E <0.001). However, several of the closest homologues of EBI-244 contained domains with moderate similarity to domain 1 and 4, along with the putative catalytic domain ( Supplementary Fig. S2 ). No sequence could be found with significant similarity to the third domain of EBI-244. The extensive predicted domain architecture is unique for GH5 family members; however, it is not unprecedented for other GH families (for example, GH2) [4] . 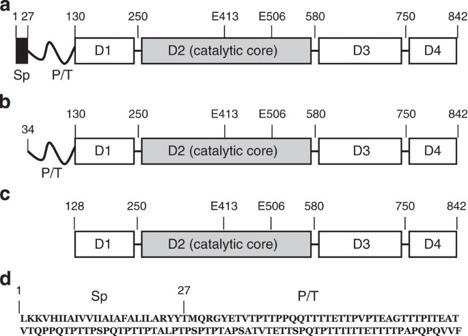Figure 4: Sequence analysis of EBI-244 enzyme. Diagrams showing predicted signal peptide/membrane anchor (Sp), Proline threonine rich low complexity region (P/T) and structural domain architecture of EBI-244. This prediction is based on HMM modelling and searching of each putative domain, as well as multiple-sequence alignments of homologous sequences (Supplementary Fig. S3is an example of a multiple alignment wherein domain boundaries are visible). Listed amino-acid positions are approximately predicted domain boundaries. (a) Diagram of predicted full-length native protein. (b) Recombinant EBI 244. (c) Recombinant EBI 244ΔN. (d) Amino-acid sequence of Signal peptide and P/T region. Figure 4: Sequence analysis of EBI-244 enzyme. Diagrams showing predicted signal peptide/membrane anchor (Sp), Proline threonine rich low complexity region (P/T) and structural domain architecture of EBI-244. This prediction is based on HMM modelling and searching of each putative domain, as well as multiple-sequence alignments of homologous sequences ( Supplementary Fig. S3 is an example of a multiple alignment wherein domain boundaries are visible). Listed amino-acid positions are approximately predicted domain boundaries. ( a ) Diagram of predicted full-length native protein. ( b ) Recombinant EBI 244. ( c ) Recombinant EBI 244ΔN. ( d ) Amino-acid sequence of Signal peptide and P/T region. Full size image The first 27 amino acids of EBI-244 likely represent a Sec-dependent signal peptide/membrane anchor ( Fig. 4 ). The PRED-SIGNAL server, designed for archaeal proteins, predicts a trans-membrane region in EBI-244 (amino acids 7–27) with the main portion of the enzyme (after amino acid 27) in the extracellular space (reliability score: 0.975). This trans-membrane region was also detected with the more general prediction servers Phobius and TMHMM. Domain 1 is followed by a region of ∼ 100 amino acids rich in Thr and Pro ( Fig. 4 ). Thr/Pro-rich regions are generally thought to be unstructured and often serve as flexible interdomain linkers in cellulases. This region is at the N-terminus and therefore not positioned between functional domains, but could provide a flexible linker extending from the membrane anchor. Cell surface-bound cellulases have been documented previously in the archaeal hyperthermophile P. horikoshii [13] . Phylogenetic analysis was carried out using the sequence of domain 2 (GH5 match) to determine its evolutionary relationship to characterized enzymes ( Fig. 5 ). The catalytic domain of EBI-244 clusters with a unique subset of TIM barrel sequences that show distant relationships to both GH families 5 and 42 in the calculated phylogenetic tree. In this analysis, three members of Family 30 formed a distant out-group, although they are assigned to the Clan A structural clade that includes the families GH5 and GH12. EBI-244 clusters with three characterized mannanases that have been classified in the GH5 family. The eight closest homologues of the EBI-244 catalytic domain include six that have a GH Pfam match (five from GH5, one from GH42), and two with no predictive matches ( E -values shown in Fig. 5 ). Given this uncertain association, the unique architecture, and the diversity of the GH5 family, it is unclear whether the sequence cluster containing the EBI-244 catalytic domain is a divergent subfamily of the GH5 family or the nucleus of a new family of glycoside hydrolases. 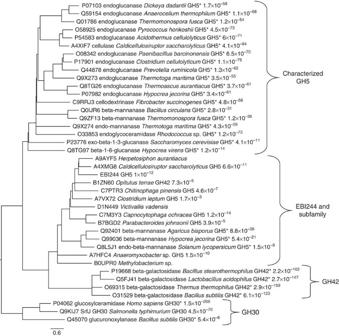Figure 5: Phylogeny of the EBI-244 protein putative catalytic domain. A phylogenetic tree was produced showing the relationship of the catalytic domain of EBI-244 to the closest characterized GH families. Tree entry information: Uniprot identifier; enzyme function (if known); organism name; Pfam hit GH family (asterisk indicated characterized enzyme in CAZy database); andE-value (where no GH is listed there was no significant Pfam hit). Figure 5: Phylogeny of the EBI-244 protein putative catalytic domain. A phylogenetic tree was produced showing the relationship of the catalytic domain of EBI-244 to the closest characterized GH families. Tree entry information: Uniprot identifier; enzyme function (if known); organism name; Pfam hit GH family (asterisk indicated characterized enzyme in CAZy database); and E -value (where no GH is listed there was no significant Pfam hit). Full size image Expression and characterization of EBI-244 EBI-244 was further characterized following its successful expression in Escherichia coli BL21 (DE3) and Rosetta cells by autoinduction [14] . Expression levels were relatively low, typically ∼ 20 μg g −1 cell pellet; however, the protein was obtained in soluble and active form after heating whole-cell extracts to 90 °C for 30 min. The purified protein was shown by N-terminal Edman sequencing to be a uniform proteolytic cleavage product truncated to Val34, determined, and, therefore, was missing the predicted signal peptide/membrane anchor ( Fig. 4b ). Recombinant EBI-244 showed endoglucanase activity on SDS–PAGE zymograms with and without refolding steps, indicating that the protein retained activity after boiling in SDS ( Supplementary Fig. S3 ). The enzyme was active on a range of high molecular weight carbohydrate substrates containing β-1,4-linked glucose, including CMC, Avicel, and filter paper ( Table 1 ). The enzyme was active toward PNP-cellobioside but inactive toward PNP-glucoside ( Table 1 ). Product analysis by fluorophore-assisted carbohydrate electrophoresis (FACE) revealed that the enzyme produces primarily cellotriose and cellotetraose from 0.33 mM cellohexaose, with a transglycosylation reaction evident from the ladder of polymers greater than cellopentaose in lanes 2–5 ( Supplementary Fig. S4 ). Table 1 The specific activity of EBI 244 endoglucanase on different substrates. Full size table Truncated versions of the protein were analysed for activity on PNP-cellobiose, CMC and Avicel to determine potential functions for each domain ( Supplementary Fig. S5 ). A truncation variant (EBI244 Δ1–127 V128M, hereafter EBI244ΔN) lacking the Thr/Pro-rich region ( Supplementary Fig. S5B ), maintained similar activity as the full-length version on the PNP-cellbioside and CMC (data not shown). This result is expected because the threonine-/proline-rich region is predicted to be a highly flexible low-complexity region. Domains 3 and 4 do not align to experimentally characterized domains, thus it is possible that these domains act as a cellulose-binding domain or function is protein–protein interactions. Truncations removing both domains 3 and 4 or just domain 4 alone ( Supplementary Fig. S5C–E ) were constructed and expressed at higher levels than the full-length protein, but were inactive against all substrates (data not shown). This result indicates that domain 3, and possibly 4 as well, is required for the enzyme to remain active, possibly due to a stabilizing effect on the enzyme. Treatment of the recombinant enzyme with proteinase K at 50 °C for 30 min, resulted in a uniform N-terminal truncation to threonine-121, determined by N-terminal Edman degradation. The proteinase treated enzyme showed similar mobility and activity to the EBI244ΔN variant (data not shown), suggesting that the remainder of the protein forms an integrated structure that is inaccessible to proteinase K at 50 °C. 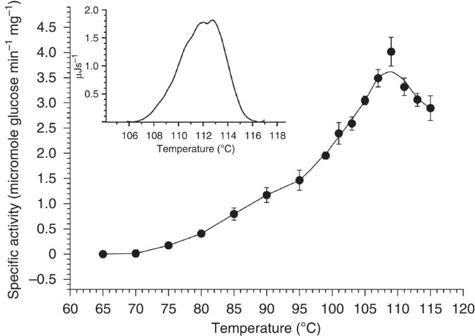Figure 6: Temperature profile of the EBI-244 enzyme. The temperature versus activity profile was measured by 20-min assay in 1% CMC in 25 mM sodium acetate buffer, pH 6.0. The products were detected by dinitrosalicylic acid reducing sugar assay and normalized to a cellobiose standard. Error for this experiment was below 15%. Inset: Differential scanning calorimetry results of enzyme from 102 to 116 °C. A dualTmwas observed at 111.5 and 113 °C. Figure 6 shows that EBI-244 had maximum activity at 109 °C and negligible activity at 70 °C when assayed against 1% CMC in 50 mM HEPPS buffer, pH 6.8. Similar results were observed with pretreated Avicel, Avicel, and Whatman No. 1 filter paper (data not shown). The enzyme had half-lives of 4.5 h in HEPPS buffer, pH 6.8, at 100 °C; 0.57 h at 105 °C in the absence of substrate ( Supplementary Fig. S6 ); and 0.17 h at 108 °C in the presence of microcrystalline cellulose (0.5% Avicel) ( Supplementary Fig. S7 ). Differential scanning calorimetry of the enzyme ( Fig. 5 , inset) showed a bifurcated transition with 2 T m 's of 111 and 113 °C. EBI-244 retained activity over a broad pH range, similar to other characterized GH5s (refs 15 , 16 ), from pH 3.5 to pH 8.0 at 95 °C, with an optimum of pH 5.5 ( Supplementary Fig. S8 ). Ionic detergents, including SDS, had little effect on enzyme activity or stability and both non-ionic and non-denaturing ionic detergents such as CHAPS-stimulated activity ( Supplementary Fig. S9 ). Figure 6: Temperature profile of the EBI-244 enzyme. The temperature versus activity profile was measured by 20-min assay in 1% CMC in 25 mM sodium acetate buffer, pH 6.0. The products were detected by dinitrosalicylic acid reducing sugar assay and normalized to a cellobiose standard. Error for this experiment was below 15%. Inset: Differential scanning calorimetry results of enzyme from 102 to 116 °C. A dual T m was observed at 111.5 and 113 °C. Full size image Given that EBI-244 remained active under high (NaCl) to near-saturating (KCl) salt conditions ( Supplementary Fig. S10 ), its activity was measured in the presence of the ionic liquids 1,3-dimethylimidazolium dimethyl phosphate (DMIM)DMP) and 1-ethyl-3-methylimidazole acetate ((EMIM)OAc), which could potentially be used to pretreat substrates like Miscanthus [17] . The concentrations tested, 25 and 50% (v/v), are well above the expected residual ionic liquid of 10–15% that may be carried over after pretreatment [18] . CMCase activity was demonstrated in zymograms, incubated at 90 °C in 25% (v/v) of either ionic liquid (pH 6.8) (data not shown). EBI-244 remained stable and active at 90 °C in 25% [DMIM]DMP ( Supplementary Fig. S10 ). Interestingly, in these assays, the enzyme's T opt decreased in the presence of ionic liquids ( Supplementary Fig. S11 ), suggesting that denaturing effects of the ionic liquids may stimulate activity at lower temperatures at which the enzyme would otherwise be inactive. Growing solely on crystalline cellulose is apparently not a simple feat, and the list of characterized organisms that grow on crystalline cellulose around 90 °C is sparse. The list includes the archaeon D. fermentans (up to 89 °C), and the bacterium C. bescii [6] , [19] . C. bescii was recently reported to grow at up to 90 °C on Avicel, filter paper and switchgrass [19] . To increase the likelihood of discovering thermophilic cellulases, we targeted microbial consortia, rather than single isolates, that would grow around 100 °C on refractory crystalline forms of cellulose. This approach, a compromise between environmental metagenomics and classical microbial isolation, resulted in the discovery of a limited archaeal enrichment capable of growing on crystalline cellulose at 90 °C, and maximally at 94 °C. Although the consortium enriched on Avicel PH-101 consisted of three strains, the closest characterized organism to the dominant member is related to I. aggregans DSM17230 (ref. 20 ), representing a divergent new species of this genus. Although similarity to characterized strains is low, environmental samples from hotsprings in Nevada and Montana have yielded 16SrDNA sequences with as close as 99% identity sequence comparison suggesting that this species may be widespread in continental geothermal systems. Single isolates from this enrichment were not possible to obtain, which was not surprising given past difficulties in isolating Ignisphaera spp. [20] It is possible that the diverse enzymes needed for lignocellulose utilization (cellulases, cellulose binding domains, CBMs, xylanases, and cellobiohydrolases) do not allow for the survival of a single isolated hyperthermophilic Archaeon given the compact genome size typically found within these organisms (<2 Mb). For example, the genome of the dominant organism in our enrichment is 1.94 Mb compared with 2.93 Mb for C. bescii . This limitation may give rise to more symbiotic relationships during cellulolytic growth at high temperatures. No archaeal cellulases from D. fermentans have been characterized to date but recently secretome and genome analysis showed several GHs coded by the bacterium C. bescii [21] . Given the limited success in finding single hyperthermophiles that can grow on crystalline cellulose, the discovery of hyperthermophilic cellulases may necessitate the broader application of enrichment driven metagenomics. The metagenome of our 90 °C consortium showed a multidomain cellulase with a high Thr/Pro N-terminal region, a core TIM barrel glycosyl hydrolase superfamily catalytic domain with low similarity to known cellulases, and uncharacterized amino-terminal domains. The cellulase, designated EBI-244, appears to be membrane-bound, a characteristic also observed for the cellulase in P. horikoshii [13] , which may be necessary to maintain the enzyme and/or the products generated in close proximity to the organism. It may also be less energy intensive to maintain enzymes on the cell surface, which would be beneficial, given the recalcitrance of the carbon. The catalytic domain of EBI-244 aligns distantly with a unique group of enzymes that are mostly uncharacterized ( Fig. 5 ). The enzymes within this group come from a variety of eukaryotic and prokaryotic organisms, including Agaricus bisporus (mushroom), Anaeromyxobacter (iron-reducing bacterium), Solanum lycopersicum (tomato plant), and Capnocytophaga ochracea (Gram-negative bacterial opportunistic pathogen). It is interesting to note that the mannanases within this subgroup all originate from eukaryotes. The bacterial and archaeal organisms from this list were isolated from diverse environments including subsurface and rice paddy sediments, the human GI tract, human faeces, the slime coat of freshwater algae, the phyllosphere or roots of plants, pine litter, and thermal springs. Although most of these organisms inhabit environments that may contain a cellulolytic substrate, most cannot use cellulose as a carbon source. Some can use cellobiose, but C. saccharolyticus and the Ignisphaera -like strain reported here are the only two that are known to be able to grow on crystalline cellulose as a sole carbon source. Among this disparate group they are also the only thermophiles. This broad diversity begs the question of why such diverse organisms have a distantly similar enzyme whereas so few organisms have one at all. It may be that the ancestral gene diverged from a manannase GH5 subfamily gene that was transferred horizontally from a eukaryote. Alternately, improved metagenomic sampling of geothermal sources could show that this cellulase clade may in fact not be rare at all, but rather is found predominantly in consortia described here. The domains composing the rest of EBI-244 generate a unique architecture for a GH5 enzyme. The truncation results indicate that deletions at the N terminus do not alter the catalytic function of the enzyme or its stability, but that domain 3 (and possibly domain 4 as well) is necessary for the catalytic domain to be functional. It is possible that these domains interact with the substrate, much like the internal cellulose-binding domain in the E4 endocellulase from Thermomonospora fusca , which not only contributes to binding but also to activity [22] . However, the inactivity of the C-terminal-truncated enzyme renders it difficult to determine whether these domains associate with the substrate or if their role is solely structural. Recombinantly expressed EBI-244 has unique properties. These include hyperthermostability (optimal activity at 109 °C, T m of 113 °C), halotolerance, resistance to ionic and non-ionic detergents, and activity in ionic liquids. The broad resilience of EBI-244 may be due to its hyperthermophilic character, not unlike other GH5 s from extremophilic organisms. Endoglucanases from P. horikoshii (EGph) and Pyrococcus furiosus had optimum temperatures of 95 and 100 °C, respectively [23] , [24] . The hyperthermophilic endoglucanases from Thermatoga maritima ( Tma Cel5A) and EGph exhibited stability in the presence of ionic liquids [25] . Recombinant Cel5A retains 44% of its activity in 15% [EMIM]OAc after 15 h whereas Pho EG retained 70% (refs. 25 , 26 ). A GH5 cellulase designated CelA 10 that is 83% similar to Cel5B from Cellovibrio japonicus , a halophile, remained active in 30% (v/v) of six different ionic liquids tested and also retained 50% and 30% activity in 4 M NaCl and 4 M KCl, respectively [26] . EBI-244 showed a similar trend of tolerance with these results from other extremophilic GH5s. In summary, this study describes the first archaeal consortium that can grow optimally, using crystalline cellulose as a carbon source at temperatures above 90 °C. Furthermore, several potential cellulases have been identified and one has been further characterized. EBI-244 is the most thermotolerant endoglucanase reported to date, and it has a unique domain architecture compared with all other hyperthermophilic GHs as well as to GH family 5 enzymes. EBI-244 also has the hallmarks of an enzyme that could enable the consortium to carry out disassembly and hydrolysis of lignocellulose, providing a new benchmark for microbial degradation of refractory lignocellulose biomass in extreme environments. Source material Sediment was removed from a pool with allochthonous decomposing wood at a site named Great Boiling Springs at 40°3945. 1 N, 119°21 59.0 W, near Gerlach, Nevada ( Fig. 1a ). A small glass jar (4 oz) was filled with sediment, topped off with spring water and sealed hot. Samples were transported on ice and long-term sample storage was carried out in anaerobic jars at 4 °C. Enrichment Strictly anaerobic microbial enrichment (90 ml) was with sediment inoculated into minimal salts medium based on DSMZ medium #516, with low yeast extract (0.2 g l −1 ) and the pulverized Miscanthus gigas (a grass, 80 μM particle size) as the primary carbon and energy source. After 3 weeks at 90 °C, a secondary enrichment with microcrystalline cellulose (Avicel Ph-101 Fluka, Ireland) was set up. The enrichment obtained on Avicel was transferred to medium containing strips of Whatman No. 3 filter paper as a sole carbon source and incubated at 90 °C until decomposition of the filter paper was observed. DNA extraction and sequencing Standard protocols for extraction of high molecular weight DNA from the Avicel enrichment using the CTAB method were followed [27] . Sequencing was done via Roche 454 titanium. Initial automated assembly was by Newbler. Automated annotation was done using a local MANATEE database and nr BLAST. In addition, further annotation was conducted through the MicrobesOnline Comparative Genomics Database. The MicrobesOnline annotation consisted of protein coding prediction using CRITICA and Glimmer3 followed by annotation using the VIMSS genome pipeline (DOE Genomes to life Program) composed of all publicly available sequence databases. Mass spectrometry Tandem mass spectrometry of peptides was conducted at the California Institute for Quantitative Biosciences Proteomics/Mass Spectrometry Core Facility. Identification of cellulase-encoding genes and gene synthesis The gene encoding the protein characterized herein was chosen because of its homology to the cellulase superfamily/glycoside hydrolase family 5 EC 3.2.1.4 as well as its similarity to a hypothetical protein from C. saccharolyticus . The gene/protein was given the designations ebi -244/EBI-244. The gene was synthesized de novo by Genscript A second version of the gene, codon optimized for expression in E. coli , was synthesized by DNA 2.0. Sequence and phylogenetic analysis Potential homologues were gathered with PSI-BLAST [28] using each putative domain of EBI-244 as the query sequence against the nr protein sequence database. The SAM software package [29] was used to build HMM's, score the potential homologue sequences, and create alignments for building new models. This method was used iteratively with each putative domain to build more general models in order to detect distant homologues. Jalview [30] was used to view and edit multiple sequence alignments. The resulting alignments allowed for approximate domain boundary determination. The phylogenetic tree was built using the SATCHMO-JS server [31] . All sequences were aligned with the Expresso server [32] to trim sequences down to only the structurally related GH domain. All characterized GH family 5 and GH family 42 sequences in the CAZy database [4] were used initially to compare with EBI-244 and its closest homologues. The size of the tree was reduced by using Jalview's remove-redundancy function, thereby also preserving the diversity of each family. The Pfam web server [2] was used to score the sequences against Pfam HMM models of the GH families. Protein expression Expression of the recombinant EBI-244 protein was routinely carried out by the autoinduction [14] . The enzyme was expressed in E. coli Rosetta cells (Invitrogen). Cells were incubated with shaking at 20 or 25 °C for 48 or 36 h, respectively. Expression was optimized in 1 l shake flask cultures, and subsequently scaled up to 17.5 l in a New Brunswick Bioflow IV fermentor. Cells were grown to an optical desnsity (OD) 550 nm of approximately 2.5–3.0 and collected by centrifugation at 6,000 g . Cells were lysed by French Pressure in 50 mM sodium phosphate buffer or 50 mM HEPPS buffer and incubated for 30 min at 90 °C. Denatured host proteins were removed by centrifugation at 8,000 g for 15 min followed by 100,000 g for 30 min. The cleared supernatant, representing a partially purified soluble fraction, was used immediately for assays or purification. Enzyme purification Native protein(s) The enrichment grown on Avicel PH-101 in a 20 l specialized fermentor was collectedted by centrifugation. The pellet, principally Avicel, was resuspended in cold (0 °C) 50 mM HEPPS buffer pH 6.8 at a rate of 10 g pellet per 40 ml and sonicated for 2 min using a Fisher Scientific 550 Sonic Dismembranator. Resuspension consisted continuous sonication for 2 min. The mixture was centrifuged (4 °C) for 15 min at 8,500 g and the supernatant was decanted. The pellet was then resuspended in HEPPS buffer and centrifugation was repeated and the supernatant decanted. The pellet was resuspended in 50 mM HEPPS/0.6% CHAPS detergent (25 °C), followed by centrifugation. The 0.6% CHAPS wash was repeated three more times and all 0.6% CHAPS fractions were pooled. The remaining washed pellet was resuspended in HEPPS buffer with 1% CHAPS and 5% cellobiose and incubated for 1 h at 90 °C, cooled to approximately ambient temperature (25 °C) and centrifuged. This wash step was repeated. The remaining pellet was resuspended in 1% SDS at 100 °C for 15 min. The CHAPS cellobiose fraction and the final fractions contained proteins including active cellulases that were presumably tightly bound to partly digested cellulose fibrils. Total activity in cell and pellet fractions was assayed by sonicating ×2 SDS–PAGE loading buffer (w/v, 2.5% SDS, 10% glycerol 60 mM Tris/HCl pH 6.8, 0.5 mM EDTA, 0.36 M 2-mercaptoethanol, 0.005% bromphenol blue) and incubated at 65 °C for 30 min before electrophoresis. Recombinant protein Clarified supernatants after heat treatment were fractionated by ammonium sulfate precipitation then buffer-exchanged on a PES membrane centrifugal concentrator (Sartorius). The protein sample was fractionated on a butyl-hydrophobic interaction column (GE Healthcare), and eluted with a linear gradient from 0.5 to 0 M ammonium sulfate in 50 mM sodium phosphate pH 6.8. Active fractions were pooled, and eluted from Q Sepharose fast flow column with a KCl gradient from 0 M to 500 mM. Zymogram visualization of cellulase activity Zymogram gels were made as standard 8% SDS–PAGE gels excepting that 0.25% medium viscosity CMC was incorporated into the gel. In the case of gradient gels, the gels were 10–15% acrylamide and contained 0.20% CMC. Standard SDS–PAGE protocols and loading buffer were used, however samples were kept at 20 °C and were not boiled before loading. The gel was agitated for 30 min in 50 mM Tris buffer pH 6.8 with 2% Triton X-100, followed by 30 min in 50 mM Tris buffer pH 6.8 incubated in 50 mM potassium phosphate pH 6.8 or 50 mM HEPPS buffer, pH 6.8 for 3 h at 90 °C, and stained with 0.5% Congo Red for 40 min. Destaining with 1 M Tris buffer pH 6.8 for 15 min at room temperature was followed by setting the dye in 1 M MgCl 2 . Cellulase assays Dinitrosalicylic acid reagent was used to detect reducing sugars at OD. Results were calibrated to standard solutions of cellobiose. Assays on CMC, Avicel, ionic liquid pretreated Avicel and Whatman No. 1 filter paper were carried out in 50 mM potassium phosphate pH 6.8 or 50 mM sodium acetate pH 5.5. Assays with high concentrations of salts or ionic liquids were carried out in phosphate buffer. Assays were usually conducted in 100 μl at T <98 °C in a thermocycler with a heated lid. Assays covering a temperature range of 100–130 °C were conducted in a silicone oil bath in silanized, heat-sealed capillary tubes (20 μl final volume). Alternative substrate assays Assays on alternative substrates described in Table 1 were done as follows Pretreated substrates were treated as previously described [9] . All cellulolytic assays for insoluble substrates were carried out in quadruplicate in a final volume of 70 μl containing 1% (w/v) substrate (glucan loading), 0.2 μM of the EBI-244 and 100 mM sodium acetate buffer, pH 5.5 at 90 °C in a thermal cycler (Applied Biosystems). Cellulase activities were measured for Avicel, Lichenan, AFEX pretreated corn stover, ionic-liquid pretreated avicel (IL-Avicel), Miscanthus (IL-Miscanthus), and corn stover (IL-corn stover). The mixtures were incubated at 90 °C for 15 h after which they were cooled to 4 °C before measuring the amount of soluble reducing sugar released using the glucose oxidase–peroxidase assay as previously described [9] . Paranitrophenol-labelled glycosides The chromogenic substrates 4-nitrophenyl-beta- D -glucopyranoside and 4-nitrophenyl-beta- D -cellobioside were utilized in 100 mM sodium acetate buffer. Sodium acetate buffer containing 4-nitrophenol was used as a standard. To compare activity at various pH levels, the following buffers were used at a buffer strength of 50 mM: pH 2.5–5.5 acetate/acetic acid, pH 6.5 MES, pH 7.5–8.5 HEPPS, pH 9.5–10.5 CAPS. All assays on PNP-substrates and standards were adjusted with an equal volume of 100 mM sodium hydroxide before recording the absorbance at 410 nm. Fluorophore assisted carbohydrate electrophoresis (FACE) Assays to determine the time course of product generation from cellopentaose and cellohexaose were performed as previously described [33] . Acccession codes: The sequence data have been deposited under accession codes JF509452 and JF509453 in the GeneBank non-redundant protein and non-redundant nucleotide databases respectively. How to cite this article: Graham, J. E. et al . Identification and characterization of a multidomain hyperthermophilic cellulase from an archaeal enrichment. Nat. Commun. 2:375 doi: 10.1038/ncomms1373 (2011).